Deregulation of translation due to post-transcriptional modification of rRNA explains whyermgenes are inducible A key mechanism of bacterial resistance to macrolide antibiotics is the dimethylation of a nucleotide in the large ribosomal subunit by erythromycin resistance methyltransferases. The majority of erm genes are expressed only when the antibiotic is present and the erythromycin resistance methyltransferase activity is critical for the survival of bacteria. Although these genes were among the first discovered inducible resistance genes, the molecular basis for their inducibility has remained unknown. Here we show that erythromycin resistance methyltransferase expression reduces cell fitness. Modification of the nucleotide in the ribosomal tunnel skews the cellular proteome by deregulating the expression of a set of proteins. We further demonstrate that aberrant translation of specific proteins results from abnormal interactions of the nascent peptide with the erythromycin resistance methyltransferase-modified ribosomal tunnel. Our findings provide a plausible explanation why erm genes have evolved to be inducible and underscore the importance of nascent peptide recognition by the ribosome for generating a balanced cellular proteome. Resistance to antibiotics is a serious clinical problem. It cripples the efficacy of drugs, especially those which have been in medical use for a considerable length of time. One of the oldest classes of antibacterials are the macrolides, which inhibit bacterial growth by binding to the nascent peptide exit tunnel (NPET) of the ribosome and interfering with protein synthesis (reviewed in refs 1 , 2 ). The prototype macrolide, erythromycin (ERY), and its modern derivatives are among the most successful antibacterials. Macrolides have been used for more than half a century for treatment of serious infections caused by a range of Gram-positive pathogens. The extensive and prolonged use of these drugs has led to the spread of resistance. One of the main resistance mechanisms is based on dimethylation of a unique adenine residue in 23S ribosomal RNA, A2058 ( Escherichia coli numbering), located in the macrolide binding site in the NPET [3] ( Fig. 1 ). This post-transcriptional modification prevents binding of the macrolides to the ribosome and renders cells resistant to very high concentrations of these drugs. The same modification confers resistance to two other classes of antibiotics, lincosamides and streptogramins B, whose binding sites in the ribosome overlap with that of macrolides [4] . The methylation of A2058 is catalysed by ERY resistance methyltransferase (Erm). The erm genes that encode this enzyme are found in the genomes of various macrolide producers, from which they have disseminated to other bacterial species, including many clinical pathogens [5] . 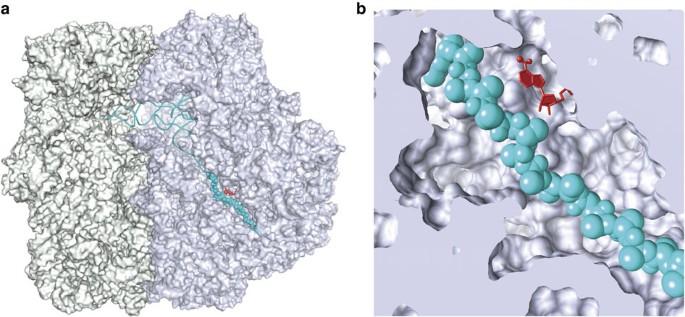Figure 1: Location of A2058 in the ribosome. (a) The structure of the bacterial ribosome with a model nascent peptide (cyan) in the exit tunnel (PDB accession numbers2WWQand2WWL(ref.38)) with the A2058 residue, the target of Erm, highlighted in red. The large ribosomal subunit is shown in pale blue and the small subunit in grey. Some rRNA and protein residues have been removed to expose the peptidyl-tRNA and the NPET. (b) The close-up view of the nascent peptide and m26A2058 in the tunnel. Two methyl groups at the exocyclic amine of A2058 (shown as balls) were added computationally. Figure 1: Location of A2058 in the ribosome. ( a ) The structure of the bacterial ribosome with a model nascent peptide (cyan) in the exit tunnel (PDB accession numbers 2WWQ and 2WWL (ref. 38 )) with the A2058 residue, the target of Erm, highlighted in red. The large ribosomal subunit is shown in pale blue and the small subunit in grey. Some rRNA and protein residues have been removed to expose the peptidyl-tRNA and the NPET. ( b ) The close-up view of the nascent peptide and m 2 6 A2058 in the tunnel. Two methyl groups at the exocyclic amine of A2058 (shown as balls) were added computationally. Full size image Early investigations of one of the first known genes of this class, ermC , led to the discovery of its inducibility: in the absence of the drug, the resistance gene was not expressed but resistance rapidly developed when cells were exposed to macrolides such as ERY [6] , [7] . The majority of more than 40 types of erm genes that are currently known show signatures of inducibility [8] , [9] , [10] , [11] ; most of the constitutive erm s appear to be merely the mutant versions of the originally inducible genes [12] , [13] , [14] . Although many examples of inducible resistance genes are now known, the drug-dependent activation of the ermC gene remains one of the most well-studied and paradigm-setting systems [3] . The molecular mechanism of ermC induction has been extensively characterized. It involves drug- and nascent peptide-controlled programmed translation arrest at the regulatory open reading frame (ORF) that leads to messenger RNA (mRNA) isomerization and activation of ermC expression [15] , [16] , [17] . It is likely that inducible expression has a key role in the rapid dissemination of erm -mediated resistance [18] . However, it remains unknown why bacteria favour erm genes to be inducible. Therefore, the driving force for evolving a complex regulatory scheme for the drug-dependent activation of expression of Erm has remained obscure. It has been speculated that expression of the erm genes could be associated with an unspecified fitness cost [19] , [20] . However, the assertion that erm expression reduces cell fitness and the reasons for the alleged fitness cost have never been experimentally demonstrated. Furthermore, it is not clear why production of Erm protein and the resulting addition of just two methyl groups with combined molecular weight of 30 Da to a site located 10 Å away from the nearest functional centre of the 2.5 million Da ribosome would be disadvantageous for bacteria ( Fig. 1 ). Here, using the prototype macrolide resistance gene ermC as a model, we demonstrate that expression of Erm notably decreases the fitness of bacteria. We show that dimethylation of an RNA nucleotide located in the NPET affects the composition of the cellular proteome by altering the level of expression of specific polypeptides. Our experiments revealed that changes in the proteome likely result from anomalous interactions of the nascent peptide with the Erm-modified exit tunnel of the ribosome. These findings provide a molecular explanation for why the erm genes evolved to be inducible. Dimethylation of A2058 by ErmC decreases bacterial fitness To test whether the expression of ErmC impacts the fitness of bacteria, we introduced the plasmid pErmCC that constitutively expresses the wild-type enzyme into the ERY-sensitive variant of the clinical Staphylococcus aureus strain USA300 ( Supplementary Fig. S1 ). Primer extension analysis ( Fig. 2a ) showed that 60% of the ribosomes in the pErmCC-transformed S. aureus are dimethylated at A2058 in 23S rRNA. These cells exhibited high resistance to ERY (minimal inhibitory concentration (MIC) >1024 μg ml −1 ) ( Table 1 ), whereas cells transformed with the empty vector (pLI50) retained unmodified A2058 ( Fig. 2a ) and remained sensitive to the drug (MIC 0.2 μg ml −1 ) ( Table 1 ). 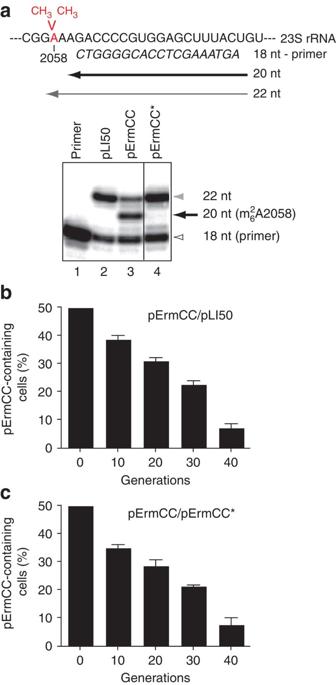Figure 2: Expression of active ErmC decreases the fitness ofS. aureus. (a) Principle of detection of A2058 dimethylation by primer extension. In the presence of dATP, dGTP, dTTP and ddCTP, reverse transcriptase extends the 18-nucleotide (nt) long primer by four nucleotides when A2058 is not modified but only by 2 nucleotides when the residue is dimethylated, because extension is impeded by the modification. The 20-nt band on the gel reflects the extent of dimethylation of A2058 in rRNA fromS. aureusUSA300 cells containing pLI50, pErmCC or pErmCC* plasmids (lanes 2–4, respectively). Lane 1 contains the labelled primer. (b,c) Growth competition betweenS. aureusUSA300 cells transformed with plasmids pErmCC and pLI50 (b), or pErmCC and pErmCC* (c). The percentage of cells expressing active ErmC was estimated by measuring the level of A2058 methylation every 10 generations for a total of ca. 40 generations. Values are the mean of three independent experiments; error bars indicate the s.d. of the mean. Figure 2: Expression of active ErmC decreases the fitness of S. aureus . ( a ) Principle of detection of A2058 dimethylation by primer extension. In the presence of dATP, dGTP, dTTP and ddCTP, reverse transcriptase extends the 18-nucleotide (nt) long primer by four nucleotides when A2058 is not modified but only by 2 nucleotides when the residue is dimethylated, because extension is impeded by the modification. The 20-nt band on the gel reflects the extent of dimethylation of A2058 in rRNA from S. aureus USA300 cells containing pLI50, pErmCC or pErmCC* plasmids (lanes 2–4, respectively). Lane 1 contains the labelled primer. ( b , c ) Growth competition between S. aureus USA300 cells transformed with plasmids pErmCC and pLI50 ( b ), or pErmCC and pErmCC* ( c ). The percentage of cells expressing active ErmC was estimated by measuring the level of A2058 methylation every 10 generations for a total of ca. 40 generations. Values are the mean of three independent experiments; error bars indicate the s.d. of the mean. Full size image Table 1 ERY MIC (μg ml −1 ) for S. aureus USA300 and RN4220 strains transformed with different plasmids. Full size table To test whether ermC expression affects cell fitness, we analysed how efficiently the pErmCC-transformed S. aureus cells competed with cells carrying the empty vector. The S. aureus /pErmCC cells were mixed in a liquid culture with equal number of S. aureus /pLI50 cells and cultures were grown for ca. 40 generations being passaged to a fresh medium after each 10-generation cycle. Changes in the ratio of the pErmCC- and pLI50-bearing cells was monitored by determining the levels of dimethylation of A2058 in the total rRNA isolated from the mixed culture. We observed that cells expressing ErmC were rapidly outcompeted by cells carrying an empty vector ( Fig. 2b ). The estimated fitness cost associated with the presence of the constitutively expressed ermC gene in the S. aureus USA300 cells was 6.5%±0.6 per generation, demonstrating that expression of ErmC has an adverse effect on cell growth in the absence of antibiotic selective pressure. Is it the production of the ErmC protein per se, or is it the catalytic activity of ErmC that accounts for the fitness cost? To address this question, we introduced the Tyr 104 -to-Ala mutation in the ErmC enzyme, which has been previously reported to inactivate its catalytic activity [21] . This mutation was engineered in the ermC gene of the pErmCC plasmid, and the resulting mutant plasmid pErmCC* was introduced into S. aureus . Western blot analysis verified that the mutant (ErmC*) protein was expressed at the level that was at least equal, if not higher, than that of wild type (ErmC) ( Supplementary Fig. S2 ). As expected, A2058 remained unmodified in the pErmCC*-transformed cells ( Fig. 2 ), which also remained sensitive to ERY ( Table 1 ), thereby verifying that the Tyr 104 -Ala mutation eliminated the methyltransferase activity of the ErmC* protein. Strikingly, in the co-growth experiment, the S. aureus /pErmCC cells were outcompeted by the S. aureus /pErmCC* cells nearly as efficiently as by the cells transformed with an empty vector ( Fig. 2c ), with the relative fitness loss of cells expressing the active enzyme of 6.3%±0.9. The deleterious effect of the expression of active ErmC was even more evident in the generally less-fit S. aureus laboratory strain RN4220 (refs 22 , 23 ), where the relative fitness cost of expressing an active enzyme versus the mutationally inactivated Erm was 7.3%±0.8. Altogether these results clearly demonstrated that the activity of the rRNA methyltransferase enzyme, rather than the mere production of the exogenous protein, is primarily responsible for the decrease in cell fitness and provided a clear biological ‘reason’ for the inducible nature of the erm genes. Chemical makeup of the NPET affects translation of specific proteins Having recognized that it is the action of the ErmC enzyme upon the ribosome that reduces fitness of S. aureus , we wanted to unravel the molecular basis of this effect. ErmC methylates 23S rRNA at the early steps of ribosome biogenesis [24] , [25] . Conceivably, the interaction of the foreign enzyme with ribosomal precursors might interfere with this process by stalling or derailing the assembly, leading to accumulation of intermediates or off-pathway products [26] . However, sucrose gradient centrifugation showed no significant differences between in the ribosomal profiles of the pErmCC- or pLI50-transformed cells ( Fig. 3a ). Furthermore, no increase in accumulation of incompletely processed rRNA in Erm-expressing cells was detected by primer extension ( Supplementary Fig. S3 ). Thus, expression of Erm seems to have little effect, if any, on assembly of the ribosome. 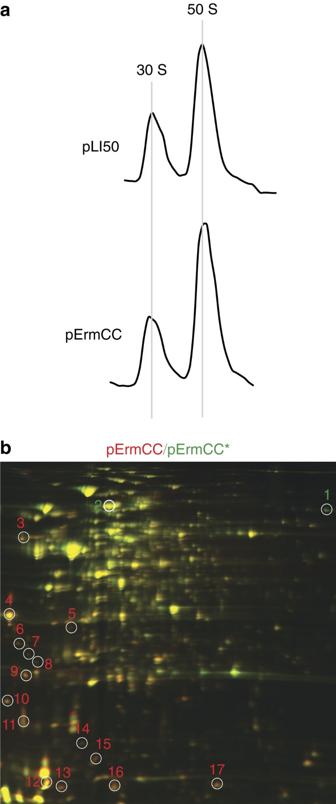Figure 3: Dimethylation of A2058 affects translation of specific polypeptides. (a) ErmC expression does not affect ribosome assembly. Sucrose gradient profiles of ribosomal subunits fromS. aureusRN4220 cells transformed with pLI50 or pErmCC plasmids. (b) Effect of dimethylation of A2058 on abundance of cellular proteins. Two-dimensional difference gel electrophoresis comparison of proteomes ofS. aureusRN4220 cells expressing active ErmC methyltransferase (pErmCC) versus cells expressing catalytically inactive Erm protein (pErmCC*) (see alsoSupplementary Fig. S4). Spots with ratios exceeding 1.5 for the pErmCC/pErmCC* and pErmCC/pLI50 pairs but being within 1.0- to 1.2-fold ratio for the pLI50/pErmCC* pair are circled and numbered from 1 to 17 (see alsoTable 2). (For spots 13 and 16 the ratios for the pLI50/pErmCC* pair exceed the 1.2-fold ratio). The spots of proteins that were expressed at lower levels in pErmCC-containing cells are numbered in green, and those expressed at a higher level are numbered in red. Figure 3: Dimethylation of A2058 affects translation of specific polypeptides. ( a ) ErmC expression does not affect ribosome assembly. Sucrose gradient profiles of ribosomal subunits from S. aureus RN4220 cells transformed with pLI50 or pErmCC plasmids. ( b ) Effect of dimethylation of A2058 on abundance of cellular proteins. Two-dimensional difference gel electrophoresis comparison of proteomes of S. aureus RN4220 cells expressing active ErmC methyltransferase (pErmCC) versus cells expressing catalytically inactive Erm protein (pErmCC*) (see also Supplementary Fig. S4 ). Spots with ratios exceeding 1.5 for the pErmCC/pErmCC* and pErmCC/pLI50 pairs but being within 1.0- to 1.2-fold ratio for the pLI50/pErmCC* pair are circled and numbered from 1 to 17 (see also Table 2 ). (For spots 13 and 16 the ratios for the pLI50/pErmCC* pair exceed the 1.2-fold ratio). The spots of proteins that were expressed at lower levels in pErmCC-containing cells are numbered in green, and those expressed at a higher level are numbered in red. Full size image An alternative possibility is that Erm-catalysed dimethylation of A2058 affects properties of the mature ribosome. As A2058 is located in the NPET ( Fig. 1 ), where functional interactions between the ribosome and the nascent peptide take place [27] , [28] , we hypothesized that changes in the chemical makeup of the tunnel surface may influence the production of certain cellular polypeptides. To explore this possibility, we used two-dimensional difference gel electrophoresis to look for possible differences in the proteomes of S. aureus cells expressing active ErmC (from pErmCC), with those of cells expressing either the inactive ErmC mutant (from pErmCC*) or no ErmC protein at all (pLI50 control). Although the majority of the proteins did not show any significant deviation in their abundance ( Fig. 3b and Supplementary Fig. S4 ), we detected several distinct protein spots whose steady-state levels in the ErmC-positive cells consistently varied 1.5- to 2.5-fold relative to both controls. Fifteen protein spots (spots 3–17) showed higher intensity in the ErmC-expressing cells, whereas two proteins (spots 1 and 2) were expressed at lower levels ( Fig. 3b , Supplementary Fig. S4 , and Table 2 ). Table 2 The difference in protein expression in cells with and without active Erm. Full size table The results of the 2two-dimensional difference gel electrophoresis analysis showed that expression of ErmC methylase, causing modification of an rRNA residue in the NPET, does not have a global effect on translation efficiency, but may lead to imbalanced translation of specific proteins, resulting in a skewed composition of the cellular proteome. Differential translation depends on the nascent peptide sequence We suspected that translation of at least some of the proteins could be directly affected by the changes in the chemical structure of an rRNA residue in the NPET. As upregulation of protein expression is more likely to be a result of a stress response (even though stress can also reduce protein expression) [29] , we focused our attention on the protein (spot 1) that was most strongly downregulated in the pErmCC-transformed cells. Mass spectrometry analysis uniquely assigned the protein in spot 1 as pyruvate oxidase (PoxB). We then examined whether the wild-type and ErmC-modified ribosomes showed any difference in translation of the poxB gene. As the nascent peptide–NPET interactions are known to affect progression of the ribosome along mRNA [17] , [30] , [31] , [32] , [33] , we hypothesized that less efficient expression of pyruvate oxidase could stem from aberrant (more- or less-prolonged) ribosome ‘dwelling’ at specific codon(s) within the gene. We examined potentially anomalous codon occupancy by analysing the difference in distribution of unmodified and Erm-dimethylated ribosomes along the poxB mRNA during its in vitro translation. Cell-free protein synthesis was carried out in a hybrid system composed of S. aureus ribosomes complemented with aminoacyl-tRNAs, and purified translation factors from E. coli . (We verified beforehand that, similar to the previously reported Bacillus subtilis/E. coli hybrid system [34] , the S. aureus ribosomes efficiently translate proteins in vitro with the assistance of E. coli factors ( Supplementary Fig. S5a )). Ribosomes were prepared either from untransformed S. aureus RN4220 cells (wild type) or from cells expressing catalytically active ErmC; 60% of ribosomes in the latter preparation were dimethylated at A2058. Direct measurements of the rate of in vitro production of PoxB were not sensitive enough to reliably detect the difference of poxB translation by unmodified or dimethylated ribosomes ( Supplementary Fig. S5b ). This is not surprising because the differential steady-state level of the protein observed in vivo could be additionally affected by translation-dependent folding and degradation, which could not be reproduced in the cell-free system. Therefore, to identify the poxB mRNA codons where the dwelling time of the Erm-modified ribosomes could be possibly different in comparison with the wild-type ribosomes, we used primer extension inhibition analysis (toeprinting) [35] . This technique has been used to analyse programmed translation arrest where prolonged occupancy by ribosomes of a specific mRNA codon inhibits progression of the reverse transcriptase producing a fairly strong complementary DNA band on the gel [17] , [36] . Although we did not anticipate stable ribosome pausing in the poxB gene and thus did not expect appearance of strong toeprinting bands, we reasoned that primer extension could still reveal subtle differences in steady-state distribution of unmodified and dimethylated ribosomes along the mRNA during in vitro translation. The analysis showed that the ribosomes with the dimethylated A2058 rRNA residue in the NPET reproducibly generated a stronger toeprint signal compared with the wild-type ribosomes, when the poxB codon Asn 118 enters the P site of the small ribosomal subunit ( Supplementary Fig. S5c ). The use of a primer annealing closer to codon 118 confirmed that the intensity of the toeprint band (representing the modified ribosomes paused at Asn 118 codon) was over 50% greater relative to the band produced by the unmethylated ribosomes ( Fig. 4a , lanes 1 and 2). This result showed that the modification of A2058 by the Erm methyltransferase leads to prolonged ribosome pausing after polymerizing 118 amino acids of the pyruvate oxidase nascent peptide. We additionally noted that at two other codons, Lys 239 and Asn 533 , methylated ribosomes produced a somewhat weaker toeprint than the wild-type ribosomes ( Supplementary Fig. S5c ). Altogether, the toeprinting data indicated that the methylation status of residue A2058 affects the rate of traversing specific codons at distinct locations of certain mRNAs. 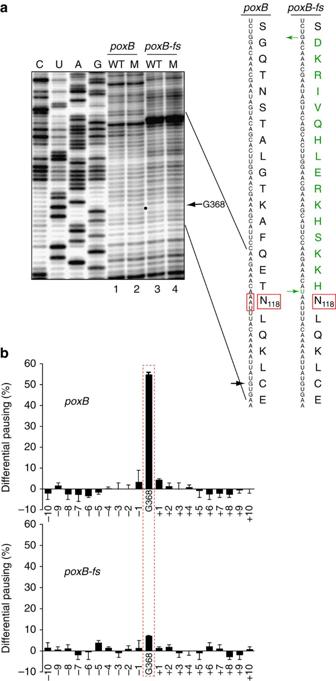Figure 4: Altered translation ofpoxBis nascent peptide dependent. (a) Toeprinting analysis of distribution of translating unmethylated (WT) or methylated (M) ribosomes along the segment of thepoxBmRNA containing the codon Asn118. The sequences of the mRNA templates encoding the wild-type PoxB (lanes 1 and 2) or the frameshift mutant PoxB-fs (lanes 3 and 4), with the altered sequence of amino-acid residues 102–117 (amino-acid residues in green), are shown on the right with the green arrows indicating the single-nucleotide deletion and insertion used to generate the mutations. The intensity of the toeprint band at thepoxBnucleotide G368 (an arrow and a dot on the gel) reflects the occupancy of the codon Asn118(boxed in red in the sequences). (b) Quantification of the differential pausing (differential intensity of the toeprint band) at G368 ofpoxBorpoxB-fsof methylated over unmethylated ribosomes. For comparison, differential intensities of bands of the 10 nucleotides preceding and following position G368 were also calculated after the background intensity was subtracted. The integrated density of five consecutive bands with seemingly similar intensities was used to normalize the data to account for potential difference in loading. Mean values were originated from three independent experiments; error bars represent the s.d. of the mean. Figure 4: Altered translation of poxB is nascent peptide dependent. ( a ) Toeprinting analysis of distribution of translating unmethylated (WT) or methylated (M) ribosomes along the segment of the poxB mRNA containing the codon Asn 118 . The sequences of the mRNA templates encoding the wild-type PoxB (lanes 1 and 2) or the frameshift mutant PoxB-fs (lanes 3 and 4), with the altered sequence of amino-acid residues 102–117 (amino-acid residues in green), are shown on the right with the green arrows indicating the single-nucleotide deletion and insertion used to generate the mutations. The intensity of the toeprint band at the poxB nucleotide G368 (an arrow and a dot on the gel) reflects the occupancy of the codon Asn 118 (boxed in red in the sequences). ( b ) Quantification of the differential pausing (differential intensity of the toeprint band) at G368 of poxB or poxB-fs of methylated over unmethylated ribosomes. For comparison, differential intensities of bands of the 10 nucleotides preceding and following position G368 were also calculated after the background intensity was subtracted. The integrated density of five consecutive bands with seemingly similar intensities was used to normalize the data to account for potential difference in loading. Mean values were originated from three independent experiments; error bars represent the s.d. of the mean. Full size image To verify the generality of this conclusion, we searched for other proteins whose translation could be affected by dimethylation of A2058. Two other differentially expressed and uniquely identified S. aureus proteins (spots 9 and 11, Fig. 3b and Supplementary Table 2 ) did not show a clear difference in the toeprinting pattern (see Discussion), which prompted us to look for other examples. Analysis of polypeptides encoded in the S. aureus genome showed that protein TenA contains the sequence Trp-Pro-Pro 108 , which has been known to slow down translation [30] . We noticed that when this protein was translated in the cell-free system, S. aureus ribosomes isolated from ErmC-expressing cells paused for a longer time at the Pro 107 codon compared with unmodified ribosomes ( Supplementary Fig. S6a ). Additionally, we tested translation of a B. subtilis protein MifM, where several translation pause sites within the sequence Asp-Ala-Gly-Ser 92 have been previously identified [37] . Again, the A2058-dimethtylated S. aureus ribosome showed a somewhat prolonged pausing at the Ser 92 codon in comparison with the wild-type ribosome ( Supplementary Fig. S6b ). Thus, it appears that dimethylation of A2058 in 23S rRNA may affect in a subtle way translation of various cellular polypeptides. The A2058 residue is located in a section of the NPET that is known to be involved in recognition of the nascent peptide [31] , [38] , [39] ( Fig. 1 ). Therefore, it is conceivable that its modification may alter interaction of the ribosome with a defined nascent peptide sequence within the tunnel. To test this idea, we introduced two compensatory frameshift mutations in the poxB mRNA, which changed the sequence of amino-acid residues Gly 102 -Thr 117 ; these 16 residues form the segment of the nascent peptide that would be located in the NPET within close proximity to A2058, when the Asn 118 codon of poxB mRNA occupies the P site of the small ribosomal subunit. Importantly, the mutations completely alter the amino-acid sequence but have minimal effect on the structure of the mRNA. Remarkably, when the mutant poxB mRNA was expressed in the hybrid cell-free translation system, wild-type and Erm-methylated ribosomes showed essentially no difference in pausing at the Asn 118 codon ( Fig. 4a , lanes 3 and 4 and Fig. 4b ). This result argues that the increased pausing of the Erm-modified ribosome at codon 118 of poxB is a consequence of aberrant interactions of the altered NPET with a specific nascent peptide structure. Even though erm s were among the first known inducible antibiotic resistance genes, the evolutionary and molecular basis for their inducibility has remained unknown. Here, we showed that expression of functionally active Erm reduces fitness of the bacterial cell possibly because dimethylation of a unique rRNA residue in the ribosomal tunnel skews expression of a subset of proteins, likely due to aberrant interactions of specific nascent peptides with the modified ribosomal exit tunnel. The fitness cost of expression of the erm gene in a clinical S. aureus strain observed in our experiments likely underestimates the cost expected to be found in nature. Expression of the ErmC from the engineered pErmCC plasmid resulted in a relatively modest degree of ribosome modification: only ca. 60% of ribosomes in the pErmCC-transformed S. aureus USA300 cells were modified ( Fig. 2a ). The higher level of ermC expression in other genetic environments [40] or the higher activity of other Erm variants [41] can produce a nearly completely modified ribosomal population, which would further increase the fitness cost. We also noted that properties of the host cell could exacerbate the competitive disadvantage of the chemically altered ribosome. Expression of catalytically active ErmC was more burdensome for the less-fit laboratory strain RN4220 (ref. 23 ), than for the clinical strain USA300. In addition, the rich laboratory media used in our experiments may further dampen the fitness difference between the wild-type and Erm-expressing cells [42] . Finally, the different structural context of A2058 in ribosomes of different species may potentially influence the fitness cost associated with its modification [43] . Therefore, in the native bacterial strains living in their natural habitats, the unnecessary expression of Erm may be highly detrimental. The considerable fitness cost of having A2058-dimethylated ribosomes would impose a strong evolutionary pressure upon bacteria to suppress expression of the erm genes in the absence of the antibiotic. Elegant mechanisms have been selected in the course of evolution of the erm genes that hinder their expression when no antibiotic is present. Remarkably, operation of these mechanisms is controlled by the modification status of A2058. In the absence of antibiotic, the unimpeded translation of the regulatory leader ORF prevents expression of the resistance gene. In the presence of the inducing antibiotic, the unmodified ribosome binds the drug and stalls at the leader ORF in a drug- and nascent peptide-dependent manner, leading to activation of erm expression. The Erm-catalysed dimethylation of A2058 not only abolishes antibiotic binding, but may also directly affect nascent peptide recognition by tunnel elements preventing translation arrest at the regulatory ORF and, thus, providing for an efficient feed-back loop that adjusts the extent of ribosome modification in response to the level of antibiotic in the environment [3] . This mechanism enables the cell to generate the minimal amount of A2058-modified ribosomes that is sufficient to maintain the adequate level of translation in the presence of the antibiotic. One of the probable explanations for the growth deficiency of Erm-expressing cells is that translation of some proteins by A2058-modified ribosomes is different compared with the ‘native’ ribosome. Two extra methyl groups at the exocyclic amine of A2058 notably change its chemical properties by increasing the hydrophobicity of the base edge and preventing the amino group from participating in hydrogen bonding interactions. The alteration in the chemical structure of the A2058 residue may significantly affect the functional properties of the NPET. A2058 is located in the NPET segment that is intimately involved in modulating translation in response to specific nascent peptides [27] , [28] , [44] . Mutations of A2058 prevent peptide-dependent ribosome stalling during translation of the regulatory SecM peptide [31] . Furthermore, dimethylation of this residue was reported to negatively affect chloramphenicol-dependent translation arrest at the ORF that controls expression of the chloramphenicol resistance gene cmlA [39] . Extrapolating these findings, it seems reasonable to expect that A2058 may also be involved in operation of more subtle regulatory circuits, where nascent peptide–ribosome interactions modulate translation elongation in a more delicate mode. The Erm-catalysed modification of A2058 could lead to deregulation of such circuits, selectively affecting expression of specific proteins. This idea is supported by our finding that dimethylation of A2058, even in a fraction of cellular ribosomes, is sufficient to notably skew production of a number of cellular polypeptides ( Fig. 3b and Table 2 ). While changes in expression of some of these proteins could be an indirect consequence of a stress response, we presented evidence that progression of the ribosome along the mRNA of at least one polypeptide, pyruvate oxidase (PoxB), is directly affected by dimethylation of A2058. PoxB expression was diminished more than twofold in cells in which only 60% of the ribosomes were modified. This change correlated with the apparent difference in the occupancy of the codons 118, 239 and 533 during in vitro translation of the poxB mRNA by A2058-modified ribosomes compared with the unmodified ribosomes. The prolonged pausing of the Erm-methylated ribosomes at codon 118 was eliminated, when the PoxB nascent peptide sequence in the NPET was mutated. This data clearly reveals that the chemical makeup of A2058 influences the ribosomal response to specific nascent peptides. It should be noted that not only slowing down, but also a needless acceleration of the evolutionary-optimized translation rate might negatively affect protein expression [45] . The observed in vitro reduced occupancy of the poxB codons Lys 239 and Asn 533 by the modified ribosome indicates a faster traverse rate that may interfere with proper protein folding and, thus, stability when the protein is expressed in the living cell [46] . It is conceivable that a similar negative effect of A2058 methylation upon accumulation of a regulatory protein (for example, a transcription repressor) may lead to upregulation of expression of some cellular polypeptides, including those present in spots 3–17 in Fig. 3b . Of note, the lack of detectable ribosome assembly defects in the Erm-expressing cells ( Fig. 3a ) argues that expression of ribosomal proteins is not significantly influenced by A2058 dimethylation. Previously, we have shown that an indigenous post-transcriptional modification of another NPET residue, A2053, is required for the proper operation of the mechanism of programmed translation arrest [47] , revealing the importance of fine structural details of the NPET for the functional recognition of the nascent peptide. Our present finding expands this observation by showing that an unwarranted modification of an rRNA residue in the NPET by an acquired rRNA methyltransferase can disrupt proper nascent peptide recognition, which leads to deregulation of expression of specific proteins. It remains to be elucidated whether A2058 functions in immediate recognition of the peptide or in relaying the signal to the peptidyl transferase center [38] , [48] . Strains and plasmids S. aureus clinical strain USA300-P23, a derivative of NARSA strain USA300-0114 (refs 49 , 50 ) rendered macrolide sensitive by curing it of plasmids 2 (30 kb) and 3 (4.3 kb), was generously provided by Dr T. Bae (Indiana University School of Medicine). Plasmid 2 contains msrA gene that encodes for the drug transporter responsible for macrolide resistance. The laboratory strain RN4220 (ref. 22 ) was used as an alternative plasmid host. The plasmid pErmCC, constitutively expressing the ermC gene under the control of the Pspac promoter [51] , was prepared by PCR amplification of the ermC gene from the pE194 plasmid [52] using primers spac-ermC-F1 and ermC-R, subsequent addition of the Pspac promoter by sequential PCRs using primer pairs spac-ermC-F2+ermC-R, spac-ermC-F3+ermC-R, spac-ermC-F4+ermC-R, ( Supplementary Table S1 ), cutting the PCR product with restriction enzymes EcoR I and Hind III, and cloning it into pLI50 shuttle cloning vector [53] opened with the same enzymes. The pErmCC* plasmid that encodes the catalytically inactive Tyr 104 -to-Ala mutant of ErmC [21] was engineered by site-directed mutagenesis of the pErmCC plasmid in which the Tyr 104 ermC codon TAT was changed to the alanine codon GCT using primer ermC(Y104A) ( Table S1 ). The plasmids expressing C-terminal His 6 -tagged wild-type (pErmCC-His 6 ) and mutant ErmC (pErmCC*-His 6 ) variants were prepared following the same strategy as described above for pErmCC and pErmCC*, except that the C-terminal His 6 -tag was introduced during PCR amplification of the ermC gene using the reverse PCR primer ermC-His-R ( Supplementary Table S1 ). Analysis of the extent of A2058 dimethylation Total RNA was isolated from S. aureus cells as previously described [54] . The extent of 23S rRNA A2058 dimethylation was assessed by primer extension using L2058 primer ( Supplementary Table S1 ) as described previously [55] with minor modifications. Specifically, 0.5 pmol of [5′- 32 P]-labelled primer L2058 was annealed to 1 μg of total RNA and extended with AMV reverse transcriptase (Roche) in the presence of 0.25 mM dTTP and 1 mM of dGTP, dATP and ddCTP. The cDNA products were resolved in a denaturing 12% polyacrylamide gel and visualized by phosphorimaging. Growth competition S. aureus USA300 or RN4220 strains transformed with pErmCC, pErmCC* or pLI50 plasmids were grown overnight in brain heart infusion (BHI) medium (BD Diagnostics) supplemented with 25 μg ml −1 of chloramphenicol. The overnight cultures were diluted to A 600 =0.05 in fresh medium containing chloramphenicol and grown at 37 °C with shaking until they reached A 600 just above 0.5. The densities of the culture were then adjusted to identical values ( A 600 =0.5). Equal culture volumes were mixed in a pair-wise manner (pErmCC/pLI50 and pErmCC/pErmCC*) and grown overnight with shaking at 37 °C. At each cycle, the cultures were diluted 1,000-fold into fresh BHI/chloramphenicol medium and grown for 24 h. Cultures were grown for a total of four passages corresponding to ca. 40 cell generations. The ratio of cells transformed with different plasmids was determined at each cycle by isolating total RNA from the co-culture and assaying the extent of dimethylation of A2058 in 23S rRNA by primer extension. The fitness cost (cost per generation) was computed using the following functions [56] : where cpg is the cost per generation, R t and S t denote the absolute number of ERY-resistant and ERY-susceptible cells at a given time t , respectively, and R t −1 and S t −1 denote the number of ERY-resistant and ERY-susceptible cells at the preceding time point, respectively. ‘ n ’ denotes the number of cell generations between time points t −1 and t . Microbiological testing MIC for ERY was determined by microbroth dilution following the standard protocol [57] . Briefly, S. aureus cells transformed with different plasmids were grown to an optical density (O.D.) of A 600 =0.5 in BHI medium supplemented with 25 μg ml −1 of chloramphenicol. Cells were then diluted to an O.D. of A 600 =0.002 and grown in 96-well plates in the presence of increasing concentrations of ERY (0.5–1024 μg ml −1 ) at 37 °C for 24 h. MIC values were defined as the minimal concentration of ERY that prevented cell growth. Preparation of S. aureus ribosomes and cell-free translation Ribosomes were isolated from S. aureus RN4220 cells (either untransformed, or transformed with pErmCC). Cells were collected by centrifugation from 1-l exponential cultures grown in BHI medium and flash frozen. Cell pellets were resuspended in 25 ml of buffer containing 10 mM Hepes–KOH (pH 7.6), 50 mM KCl, 10 mM Mg(OAc) 2 , 7 mM β-mercaptoethanol, 0.1 mg ml −1 lysostaphin (Sigma-Aldrich) and disrupted by two passes through French press at 20,000 psi. Cell debris was removed by centrifugation at 20,000 g for 30 min. Ribosomes were then purified from the cell lysates by chromatography on the HiTrap Butyl FF resin (GE Healthcare) [58] . Status of A2058 modification was verified by primer extension analysis of the rRNA isolated by phenol extraction from the ribosome preparation. In vitro translation and toeprinting were carried out essentially as previously described [17] with some modifications. Specifically, in vitro transcription/translation was performed in a 5-μl reaction using the E. coli Δribosome PURExpress kit (New England Biolabs), which lacks ribosomes, supplemented with 10 pmoles of purified S. aureus ribosomes. Except for reducing the reaction volume down to 5 μl and using heterologous ribosomes, the reactions were assembled following the manufacturer’s protocol. DNA templates were prepared by PCR amplification of S. aureus genes with their ribosome-binding sites, using genomic DNA prepared from the RN4220 strain as template (primers are listed in Supplementary Table S1 ). The T7 promoter required for in vitro transcription was introduced on the forward PCR primer. The control dhfr template was provided with the PURExpress kit. The bands in the toeprinting gels were quantified using ImageJ software ( http://rsbweb.nih.gov/ij/ ). For introducing compensatory frameshift mutations, the poxB gene was first 3′-truncated and Asp 137 codon was mutated to a stop codon (TAA) using primers T7-poxB and poxB(short)-R ( Supplementary Table S1 ). The compensatory frameshift mutations that changed the sequence of the nascent peptide encoded in codons 102–117 in the poxB gene were introduced by two-step PCR using primers T7-poxB and poxB.F-R in the first PCR reaction followed by PCR with primers T7-poxB and poxB(short)-R. Analysis of ribosomal subunits and precursors The ribosomal subunits from exponentially growing S. aureus RN4220 cells transformed with pLI50 and pErmCC were analysed as previously described [59] . Briefly, exponentially growing cells were pelleted and resuspended in 400 μl of buffer S: 10 mM Tris–HCl (pH 7.8), 1 mM Mg diacetate, 50 mM NH 4 Cl, 2 mM β-mercaptoethanol, supplemented with lysostaphin (50 μg ml −1 ) (Sigma) and RNase inhibitor (100 U ml −1 ) (Thermo Scientific). Cells were lysed by incubation for 20 min at room temperature. Two units of RQ DNase (Promega) were added to each sample, and after 5 min of incubation at room temperature, samples were spun for 10 min at 21,000 g . Lysates were loaded onto 10–40% sucrose gradient prepared in buffer S, centrifuged in the SW41 rotor at 24,500 r.p.m for 18 h at 4 °C and then fractionated. Presence of ribosomal precursors was analysed by primer extension carried out using total RNA isolated from pLI50- or pErmCC-transformed RN4220 cells. The primers SaS20 and SaL20 annealing close to the 5′ ends of 16S and 23S rRNA, respectively, were used in the analysis ( Supplementary Table S1 ). Proteomics S. aureus RN4220 transformed with pErmCC, pErmCC* or pLI50 plasmids were grown overnight in BHI medium supplemented with 25 μg ml −1 chloramphenicol. The overnight cultures were diluted to an O.D. of A 600 =0.05 in fresh chloramphenicol containing medium and grown at 37 °C with shaking to an O.D. of 0.5. Cells were pelleted, washed twice with PBS buffer and flash frozen. Protein extraction, labelling and two-dimensional gel electrophoresis was performed by Applied Biomics, Hayward, CA, using a linear pH gradient 4–7 in the first dimension [60] . Gels were scanned using Typhoon TRIO (GE Healthcare). The images were analysed by Image Quant (GE Healthcare) and DeCyder software (GE Healthcare). Spots with consistent ratios below 0.67 or above 1.5 for the pLI50/pErmCC and pErmCC*/pErmCC pairs, but within the 0.83–1.2 range for the pLI50/pErmCC* pair, were cut from the gel using a spot picker robot. Proteins were extracted and their tryptic digests analysed by mass spectrometry at the proteomics facility of the University of Illinois at Chicago. Analysis of ErmC expression S. aureus cells (RN4220) transformed with pErmCC-His 6 or pErmCC*-His 6 plasmids were grown in 5 ml BHI medium supplemented with 25 μg ml −1 chloramphenicol. When cultures reached an O.D. of A 600 =0.5, cells were pelleted and resuspended in 200 μl of the buffer: 10 mM Tris–HCl (pH7.5), 30 mM MgCl 2 , 30 mM NH 4 Cl, containing 0.5 mg ml −1 of lysostaphin (Sigma-Aldrich). Lysis was completed by incubating the cell suspensions at 37 °C for 1 h. Samples with 25 μg of protein (ca. 20 μl of the lysate) were loaded onto 4–20% Mini-PROTEAN TGX gel (Bio-Rad) and resolved by electrophoresis. Proteins were then transferred to a polyvinylidene difluoride membrane and probed using anti-His 6 HRP-coupled antibodies (Thermo Scientific). As a loading control, equal amounts of lysates were run on a separate gel and stained with Coomassie G-250. How to cite this article: Gupta, P. et al. Deregulation of translation due to post-transcriptional modification of rRNA explains why erm genes are inducible. Nat. Commun. 4:1984 doi: 10.1038/ncomms2984 (2013).